IL-10-producing intestinal macrophages prevent excessive antibacterial innate immunity by limiting IL-23 synthesis Innate immune responses are regulated in the intestine to prevent excessive inflammation. Here we show that a subset of mouse colonic macrophages constitutively produce the anti-inflammatory cytokine IL-10. In mice infected with Citrobacter rodentium , a model for enteropathogenic Escherichia coli infection in humans, these macrophages are required to prevent intestinal pathology. IL-23 is significantly increased in infected mice with a myeloid cell-specific deletion of IL-10, and the addition of IL-10 reduces IL-23 production by intestinal macrophages. Furthermore, blockade of IL-23 leads to reduced mortality in the context of macrophage IL-10 deficiency. Transcriptome and other analyses indicate that IL-10-expressing macrophages receive an autocrine IL-10 signal. Interestingly, only transfer of the IL-10 positive macrophages could rescue IL-10-deficient infected mice. Therefore, these data indicate a pivotal role for intestinal macrophages that constitutively produce IL-10, in controlling excessive innate immune activation and preventing tissue damage after an acute bacterial infection. Interleukin 10 (IL-10) is an immunoregulatory cytokine that limits mucosal immune responses and minimizes immunopathology. Indeed, mutations in the interleukin 10 (IL-10) receptor gene ( Il10r ) were found in some patients with early-onset colitis [1] , [2] . Similarly, mice deficient for IL-10 ( Il10 − / − ) or IL-10R ( Il10rb − / − ) developed spontaneous inflammation of the large intestine, a process that was T-cell dependent and dominated by a pathogenic T helper type 1 and type 17 (Th1 and Th17) immune responses [3] , [4] , [5] . A number of cell types can produce IL-10, including lymphocytes, monocytes, macrophages, mast cells, keratinocytes and intestinal epithelial cells. In several colitis models, the role of T-cell-derived IL-10 has proven to be central [6] , [7] , [8] , and in fact, mice with a conditional deletion of IL-10 in the CD4 + T-cell subset develop spontaneous inflammation of the intestine, as do those with a deletion in regulatory T cells (Treg) mediated by a Foxp3 driven Cre (refs 9 , 10 ). However, we found IL-10 from macrophages plays an indispensable role in the maintenance of Foxp3 expression by Treg and their function in mice with colitis [11] . Despite this, mice with a conditional deletion of IL-10 or IL-10R in myeloid cell subsets [12] , [13] , or of IL-10 specifically in macrophages [14] , did not spontaneously develop aggressive colitis, although they were susceptible to excessive inflammation following systemic LPS exposure [12] , [13] . These data suggest that myeloid cell derived IL-10 might have a pivotal role in controlling mucosal immune responses after bacterial infection. In the context of acute mucosal infections, the lack of IL-10 could be protective because of an enhanced inflammatory response with increased IL-12, tumour necrosis factor (TNF) and other cytokines [15] , [16] , [17] , [18] , [19] , [20] . However, the absence of IL-10 also could lead to excessive inflammation [17] , [21] , [22] , [23] . Therefore, in the context of acute bacterial infection of the intestine, it remains to be determined which cell type(s) produce IL-10, if IL-10 is protective or harmful, and which pathways are activated or inhibited by IL-10 secretion. To explore these issues, we have analysed mice with cell type-specific deletion of Il10 that were infected with Citrobacter rodentium ( C. rodentium ). This is a Gram-negative bacterium that is considered a model for enteropathogenic and enterohemorrhagic Escherichia coli infections in humans. C. rodentium causes attaching and effacing mechanism of epithelial infection, leading to intestinal inflammation and diarrhoea. The bacteria normally are cleared in wild-type mice due to the actions of innate and adaptive immunity and the intestinal inflammation ultimately resolves [24] , [25] , [26] . Here we show that a unique subset of macrophages in the colonic lamina propria that constitutively produces IL-10 plays a critical role in preventing excessive inflammation following acute bacterial infection by limiting innate immunity, and that a major pathway by which IL-10 acts is through controlling IL-23 production. Myeloid cell IL-10 is important for survival from C. rodentium To assess the function of IL-10 in regulating mucosal immune responses after intestinal bacterial challenge, we used Il10 − / − , Il10rb − / − and wild-type (wt) recipient mice that were infected with a sublethal dose of C. rodentium by oral gavage. The onset and severity of colitis in Il10 − /− mice is strongly influenced by the genetic background [3] , and we used mice on the C57BL6/J background that are more protected from inflammation under steady-state conditions. Indeed, none of the groups developed spontaneous colitis in our mouse colony ( Supplementary Fig. 1 ). However, we found that all Il10 −/− and Il10rb −/− mice died 7–12 days after infection, whereas all wt mice survived ( Fig. 1a ). At day 6 after infection, Il10 −/− and Il10rb −/− mice showed severe colonic inflammation, characterized by epithelial cell destruction, infiltration of mononuclear cells ( Supplementary Fig. 1 ). These indicate that the role of IL-10 in modulating the initial mucosal immune response against C. rodentium is indispensable for survival and mucosal damage. 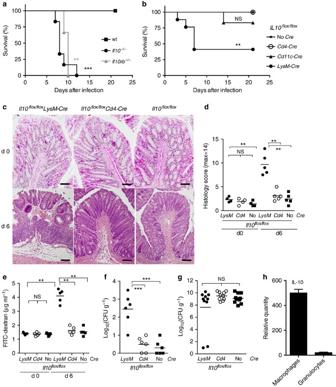Figure 1: Myeloid cell-derived IL-10 is crucial for survival afterCitrobacter rodentiuminfection. (a)Il10−/−(black circle),Il10rb−/−(grey triangle) and C57BL/6J (black square) mice or (b)Il10flox/floxLysM-Cre(black circle),Il10flox/floxCd4-Cre(open circle),Il10flox/floxCd11c-Cre(black triangle) andIl10flox/flox(black square) mice were infected orally withC. rodentiumand survival was monitored. (a) Two independent experiments with 6 mice per group and (b) 3 independent experiments with 12–17 mice per group are presented. (a,b) Log-rank test, **P<0.01, ***P<0.001 (c,d) inflammation of middle colon was assessed by histology before and 6 days after infection. Scale bars, 100 μm. (e) Epithelial barrier permeability was determined before and 6 days after infection. (f,g) Titres ofC. rodentiuminfspleen andgfaeces were quantified 6 days of infection. (e–g) Each symbol represents a measurement from a single mouse. Student’st-test, **P<0.01, ***P<0.001 (h) Analysis ofIl10mRNA in macrophages or granulocytes at day 3 after infection. Results were representative of two independent experiments. NS, non significant. Figure 1: Myeloid cell-derived IL-10 is crucial for survival after Citrobacter rodentium infection. ( a ) Il10 −/− (black circle), Il10rb −/− (grey triangle) and C57BL/6J (black square) mice or ( b ) Il10 flox/flox LysM-Cre (black circle), Il10 flox/flox Cd4-Cre (open circle), Il10 flox/flox Cd11c-Cre (black triangle) and Il10 flox/flox (black square) mice were infected orally with C. rodentium and survival was monitored. ( a ) Two independent experiments with 6 mice per group and ( b ) 3 independent experiments with 12–17 mice per group are presented. ( a , b ) Log-rank test, ** P <0.01, *** P <0.001 ( c , d ) inflammation of middle colon was assessed by histology before and 6 days after infection. Scale bars, 100 μm. ( e ) Epithelial barrier permeability was determined before and 6 days after infection. ( f , g ) Titres of C. rodentium in f spleen and g faeces were quantified 6 days of infection. ( e – g ) Each symbol represents a measurement from a single mouse. Student’s t- test, ** P <0.01, *** P <0.001 ( h ) Analysis of Il10 mRNA in macrophages or granulocytes at day 3 after infection. Results were representative of two independent experiments. NS, non significant. Full size image To identify which cell type(s) produce the IL-10 that is essential for host protection, we analysed mice with cell type-specific deletions of the Il10 gene. These included Il10 flox/flox LysM-Cre , with deletion targeted primarily to CD11b + myeloid cells, including macrophages, monocytes and neutrophils, Il10 flox/flox Cd4-Cre targeting mostly CD4 + T cells, and Il10 flox/flox Cd11c-Cre mice, which acts predominantly in dendritic cells (DCs). We used Il10 flox/flox Cre − ( Il10 flox/flox ) littermates for controls. We found that Il10 flox/flox LysM-Cre mice started to die early after C. rodentium infection, with less than half surviving beyond day 7. In contrast, most of the Il10 flox/flox Cd11c-Cre and all of the Il10 flox/flox Cd4-Cre recipients survived to 21 days after infection ( Fig. 1b ). The average histology scores of each group were similar before C. rodentium infection. With the dose of bacteria we used, at day 6 we observed mild inflammation in Il10 flox/flox Cd4-Cre and Il10 flox/flox recipients, manifested by epithelial cell hyperplasia and some cellular infiltration. However, Il10 flox/flox LysM-Cre recipients, most of which survived to day 6, developed significantly more severe colonic inflammation, characterized by epithelial cell destruction, infiltration of mononuclear cells and submucosal oedema in the large intestine ( Fig. 1c,d ). In parallel with this, we found increased colonic epithelial permeability and bacterial dissemination to the spleen after infection in Il10 flox/flox LysM-Cre recipients ( Fig. 1e,f ). Despite this, bacterial numbers in the faeces of Il10 flox/flox LysM-Cre recipients at day 6 after bacterial challenge were similar compared with Il10 flox/flox Cd4-Cre and Il10 flox/flox mice ( Fig. 1g ). These data suggest intestinal epithelial cell destruction by excessive mucosal immune responses after infection in Il10 flox/flox LysM-Cre recipients probably contributed to bacterial dissemination and lethality. Macrophages are the principal IL-10-producing cells We assessed the effectiveness and specificity of the deletion of Il10 in the various cell populations by measuring the decrease in Il10 mRNA at steady state. Indeed, we detected a decrease of ∼ 90% in Il10 mRNA transcripts in the CD11c int CD11b + macrophage population from the colon of Il10 flox/flox LysM-Cre mice compared with Il10 flox/flox controls, with little decrease in CD11c + CD11b − cells or CD4 + T cells ( Supplementary Fig. 2 ). Similarly, we detected a specific and nearly complete loss of Il10 transcripts in CD4 + T cells in Il10 flox/flox Cd4-Cre mice and a similar decrease in the CD11c + CD11b − population in Il10 flox/flox Cd11c-Cre mice . There also was a 15–20% decrease in Il10 mRNA in the CD11c int CD11b + population in Il10 flox/flox Cd11c-Cre mice ( Supplementary Fig. 2 ). The intermediate level of CD11c expression by macrophages in the CD11c int CD11b + population likely is responsible for the incomplete disruption of IL-10 expression and the preservation of protective function in the Il10 flox/flox Cd11c-Cre strain. Therefore, we conclude that the absence of a strong effect on the survival and inflammation in the Il10 flox/flox Cd4-Cre and Il10 flox/flox Cd11c-Cre strains is not due to the inefficient removal of the Il10 gene. Because the LysM promoter drives Cre recombinase expression in macrophages, monocytes and neutrophils, we determined which of these cell types produced IL-10 after infection. Consistent with a recent report [20] , IL-10 mRNA was most highly expressed in CD11b + CD11c int macrophages, which also express F4/80 and MHC class II, but was undetectable in granulocytes ( Fig. 1h ) in the large intestine. Therefore, the reduced survival in Il10 flox/flox LysM-Cre mice is very likely due to the loss of IL-10 production by macrophages. A significant proportion of macrophages were IL-10 competent, GFP + cells in the large intestine before infection. By flow cytometry, these cells were more frequent in the colon compared with the small intestine ( Supplementary Fig. 3a ). When analysed by immunohistology, both the GFP + (IL-10 + ) and GFP − (IL− 10 − ) macrophages were scattered from the top of the villi to the crypt in both the small and the large intestine ( Supplementary Fig. 3b ). This population is maintained through day 6 of infection ( Supplementary Fig. 4 ), although the frequency tended to decrease. To confirm that IL-10-producing macrophages regulate mucosal innate immune responses independently of adaptive immunity, we analysed intestinal inflammation triggered by C. rodentium using Rag −/− and Il10 −/− Rag −/− mice. Il10 −/− Rag −/− mice had more severe mortality and severe colonic inflammation at day 6 after infection compared with Rag −/− mice ( Supplementary Fig. 5 ). Together, these data suggest that macrophage-derived IL-10 plays a nonredundant role in limiting the innate mucosal immune responses against intestinal infection with C. rodentium . Macrophage IL-10 regulates myeloid cell recruitment to the colon To determine if macrophage-derived IL-10 regulates inflammatory cell recruitment to the large intestine after C. rodentium infection, we examined the kinetics of cell accumulation in the colon lamina propria in Il10 flox/flox LysM-Cre , Il10 flox/flox Cd4-Cre and Il10 flox/flox recipients during C. rodentium infection, and we characterized the infiltrating cell types by flow cytometric analysis. The total cell number in the colon lamina propria was comparable in all the groups before C. rodentium injection, and CD11b + Ly6G − Ly6C high monocytes were undetectable ( Fig. 2a ). Six days after infection, we detected a significant increase in total cell numbers in Il10 flox/flox LysM-Cre mice compared with Il10 flox/flox Cd4-Cre and Il10 flox/flox recipients, and the population in the large intestine lamina propria consisted mainly of CD11b + Ly6G − Ly6C high monocytes and CD11b + Ly6G high Ly6C low granulocytes ( Fig. 2a ). There was no increase in CD4 + T cells in any of these groups at this early time point ( Fig. 2a ). 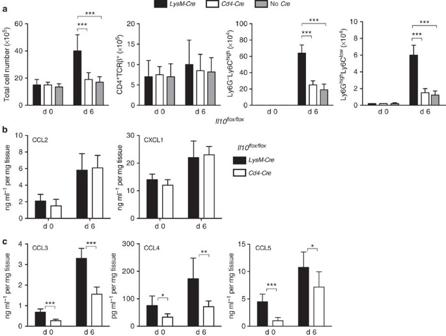Figure 2: Macrophage IL-10 regulates myeloid cell recruitment to the colon. Il10flox/floxLysM-Cre(black),Il10flox/floxCd4-Cre(white) andIl10flox/flox(grey) mice were analysed before and at day 6 afterC. rodentiuminfection. (a) Lamina propria cells were isolated at the indicated times and total cell numbers were counted. Frequencies of CD4+T cells (CD4+TCRβ+), monocytes (Ly6G−Ly6Chigh) and granulocytes (Ly6GhighLy6Clow) were measured by flow cytometry and cell numbers were calculated according to the respective total cell number. Cell numbers are presented as averages and s.d. from nine mice per group from three independent experiments. (b,c) At the indicated time points, 3-mm fragments of the middle colon ofIl10flox/floxLysM-Cre(black),Il10flox/floxCd4-Cre(white) mice were cultured for 24 h. Chemokine production was measured in the supernatants by Multiplex cytokine assay and normalized to the weight of the corresponding tissue fragments. Data are presented as averages with s.d. from two independent experiments with six mice in each group. Student’st-test, *P<0.05, **P<0.01, ***P<0.001. Figure 2: Macrophage IL-10 regulates myeloid cell recruitment to the colon. Il10 flox/flox LysM-Cre (black), Il10 flox/flox Cd4-Cre (white) and Il10 flox/flox (grey) mice were analysed before and at day 6 after C. rodentium infection. ( a ) Lamina propria cells were isolated at the indicated times and total cell numbers were counted. Frequencies of CD4 + T cells (CD4 + TCRβ + ), monocytes (Ly6G − Ly6C high ) and granulocytes (Ly6G high Ly6C low ) were measured by flow cytometry and cell numbers were calculated according to the respective total cell number. Cell numbers are presented as averages and s.d. from nine mice per group from three independent experiments. ( b , c ) At the indicated time points, 3-mm fragments of the middle colon of Il10 flox/flox LysM-Cre (black), Il10 flox/flox Cd4-Cre (white) mice were cultured for 24 h. Chemokine production was measured in the supernatants by Multiplex cytokine assay and normalized to the weight of the corresponding tissue fragments. Data are presented as averages with s.d. from two independent experiments with six mice in each group. Student’s t -test, * P <0.05, ** P <0.01, *** P <0.001. Full size image Because myeloid cell infiltrates were increased in infected Il10 flox/flox LysM-Cre mice, we tested if chemokines that would attract these cells were also increased. Because Il10 flox/flox Cd4-Cre and Il10 flox/flox recipients were similar in survival and degree of inflammation, we compared Il10 flox/flox LysM-Cre mice with Il10 flox/flox Cd4-Cre mice. Although CCL2 and CXCL1, known to recruit monocytes and granulocytes, respectively, were similar between Il10 flox/flox LysM-Cre mice and Il10 flox/flox Cd4-Cre mice ( Fig. 2b ), other chemokines that recruit monocytes and neutrophils, including CCL3, CCL4 and CCL5, were significantly increased in colon fragment culture supernatants from Il10 flox/flox LysM-Cre mice ( Fig. 2c ). This was true even before C. rodentium infection ( Fig. 2c ), although this increased level before infection apparently was not sufficiently high to recruit monocytes and granulocytes and cause detectable inflammation. These data suggest that macrophage-derived IL-10 regulates the chemokine-dependent recruitment of monocytes and granulocytes to the large intestine during intestinal bacterial infection. Increased pro-inflammatory cytokines in Il10 flox/flox LysM-Cre mice We examined if the increased colitis in C. rodentium- infected Il10 flox/flox LysM-Cre mice was associated with the excessive production of pro-inflammatory cytokines using a Bio-Plex multicytokine assay. As illustrated ( Fig. 3 ), IL-10 production was reduced before infection and early after infection in Il10 flox/flox LysM-Cre compared with Il10 flox/flox Cd4-Cre mice, suggesting that the majority of IL-10 in the colon under these conditions is produced by macrophages. Conversely, the production of TNF and IL-12p40 was increased in Il10 flox/flox LysM-Cre recipients in colon fragment cultures before and more strongly during infection, while IL-6 and interferon γ levels were comparable. We used a different method, enzyme-linked immunosorbent assay (ELISA), to explore the expression of IL-12 family cytokines further. We detected a striking increase in IL-23p19 by day 6 after infection in Il10 flox/flox LysM-Cre mice. However neither IL-23 nor IL-12p70 were significantly increased in Il10 flox/flox LysM-Cre before infection, suggesting that IL-12p40 monomers or dimers, known to be produced in other contexts [27] , [28] , likely were produced in the intestine under the lack of macrophage-derived IL-10, although the function of IL-12p40 homodimers is uncertain. 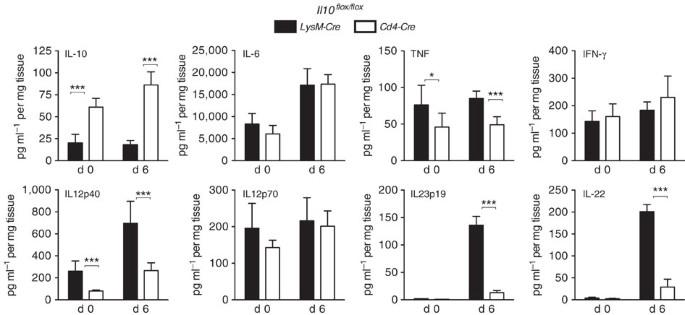Figure 3: Increased pro-inflammatory cytokines in the large intestine inIl10flox/floxLysM-Cremice. Il10flox/floxLysM-Cre(black) andIl10flox/floxCd4-Cre(white) mice were analysed at day 0 or day 6 afterC. rodentiuminfection. At the indicated time points, 3-mm fragments of the middle colon were cultured for 24 h. Cytokine production was measured in the supernatants by Multiplex or ELISA and normalized to the weight of the corresponding tissue fragments. Averages and s.d. from two independent experiments with six mice in each group are presented. Student’st-test, *P<0.05, ***P<0.001. IFN-γ , interferon γ. Figure 3: Increased pro-inflammatory cytokines in the large intestine in Il10 flox/flox LysM-Cre mice. Il10 flox/flox LysM-Cre (black) and Il10 flox/flox Cd4-Cre (white) mice were analysed at day 0 or day 6 after C. rodentium infection. At the indicated time points, 3-mm fragments of the middle colon were cultured for 24 h. Cytokine production was measured in the supernatants by Multiplex or ELISA and normalized to the weight of the corresponding tissue fragments. Averages and s.d. from two independent experiments with six mice in each group are presented. Student’s t- test, * P <0.05, *** P <0.001. IFN-γ , interferon γ. Full size image It has been reported that IL-23 induces IL-22 production from innate lymphoid cells [29] , [30] . Indeed, consistent with the significant increase in IL-23 by day 6 after infection, in colonic fragment cultures from infected Il10 flox/flox LysM-Cre mice, we detected a profound increase in IL-22 production as well ( Fig. 3 ). Macrophage IL-10 influences mortality through the regulation of IL-23p19 We assessed if IL-10 acts on the IL-23p19-producing cells activated by C. rodentium . It has been reported IL-23 is produced by macrophages and DCs [29] , [31] , [32] . To determine the dominant source of IL-23-producing cells, we sorted CD11b + CD11c int F4/80 + colonic macrophages and CD11b − CD11c + F4/80 − DCs from two strains of IL-10-deficient mice at day 6 after infection, and compared the Il23p19 , Il12p40 and Il12p35 mRNA transcripts. Macrophages tended to have higher amounts of each of these transcripts, but importantly, mice with a LysM Cre -mediated deletion of IL-10 had increased amounts of Il23p19 and Il12p40 mRNA, while Il12p35 mRNA transcripts were similar to mice with a CD4 Cre-mediated deletion ( Fig. 4a ). To determine if IL-10 by macrophages regulates IL- 23 production, we sorted GFP + (IL-10 + ) and GFP − (IL-10 − ) macrophages from Il10 gfp mice before and after C. rodentium infection. We detected significantly increased amounts of Il23p19 mRNA in GFP − macrophages compared with those in GFP + cells after infection, suggesting an autocrine role for IL-10 in the reporter positive cells. There were very few Il23p19 mRNA transcripts in either type of macrophages before infection, but even in the GFP + macrophages there was a small increase in Il23p19 mRNA following the exposure to C. rodentium ( Fig. 4b ). We also sorted macrophages from the large intestine of mice with a germline Il10 deficiency at day 3 after infection, cultured them with or without the addition of recombinant IL-10, and analysed the supernatants by ELISA. Exogenous IL-10 completely abrogated IL-23p19 production by colonic macrophages from infected mice; but had little effect on the IL-6 production ( Fig. 4c ). IL-12p70 was undetectable at this time, with or without the addition of IL-10 (data not shown). These data suggest that IL-10 might inhibit IL-23 production in vivo following infection, in part by acting directly on the IL-23-producing macrophages. 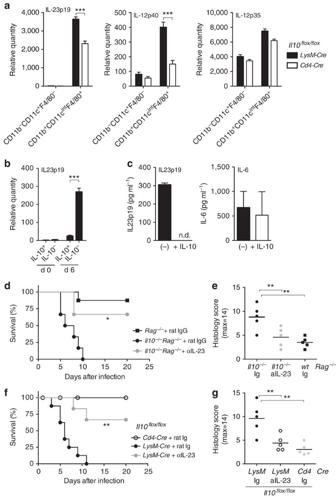Figure 4: Macrophage-derived IL-10 influences mortality through regulation of IL-23p19. (a) Analysis of gene expression by reverse transcription PCR (RT-PCR) in sorted CD11b−CD11c+F4/80−DC or CD11b+CD11cintF4/80+macrophages from large intestines inIl10flox/floxLysM-CreorIl10flox/floxCd4-Cremice at day 6 afterC. rodentiuminfection. Averages and s.d. from two independent experiments with six mice in each group are shown. (b) Analysis ofIl23p19mRNA transcripts by RT-PCR in large intestine lamina propria macrophages, including GFP+(IL-10+) and GFP−(IL-10−), sorted from five to eightIl10gfpmice before and after 6 days afterC. rodentiuminfection. These data are from two independent experiments. (c) Large intestine lamina propria macrophages were sorted from five to eight infectedIl10−/−Rag−/−mice and cultured for 24 h in the absence (black bars) or presence (white bars) of 100ng ml−1recombinant mouse IL-10. Supernatants were analysed for IL23p19 and IL-6 by ELISA. These data are from 2–3 independent experiments. (d,e)Il10−/−Rag−/−andRag−/−mice or (f,g)Il10flox/floxLysM-CreandIl10flox/floxCd4-Cremice were infected withC. rodentium. (d–g) At the time of infection, 100 μg anti-IL-23 or rat IgG were injected per mouse intravenously. (d,f) Survival curve and (e,g) histology score from middle colon at day 6 after infection are shown. These are from two independent experiments with 3–4 mice per group. Student’st-test, *P<0.05, **P<0.01, ***P<0.001. Figure 4: Macrophage-derived IL-10 influences mortality through regulation of IL-23p19. ( a ) Analysis of gene expression by reverse transcription PCR (RT-PCR) in sorted CD11b − CD11c + F4/80 − DC or CD11b + CD11c int F4/80 + macrophages from large intestines in Il10 flox/flox LysM-Cre or Il10 flox/flox Cd4-Cre mice at day 6 after C. rodentium infection. Averages and s.d. from two independent experiments with six mice in each group are shown. ( b ) Analysis of Il23p19 mRNA transcripts by RT-PCR in large intestine lamina propria macrophages, including GFP + (IL-10 + ) and GFP − (IL-10 − ), sorted from five to eight Il10 gfp mice before and after 6 days after C. rodentium infection. These data are from two independent experiments. ( c ) Large intestine lamina propria macrophages were sorted from five to eight infected Il10 −/− Rag −/− mice and cultured for 24 h in the absence (black bars) or presence (white bars) of 100ng ml −1 recombinant mouse IL-10. Supernatants were analysed for IL23p19 and IL-6 by ELISA. These data are from 2–3 independent experiments. ( d , e ) Il10 −/− Rag −/− and Rag −/− mice or ( f , g ) Il10 flox/flox LysM-Cre and Il10 flox/flox Cd4-Cre mice were infected with C. rodentium . ( d – g ) At the time of infection, 100 μg anti-IL-23 or rat IgG were injected per mouse intravenously. ( d , f ) Survival curve and ( e , g ) histology score from middle colon at day 6 after infection are shown. These are from two independent experiments with 3–4 mice per group. Student’s t -test, * P <0.05, ** P <0.01, *** P <0.001. Full size image To elucidate if increased IL-23 production in the absence of IL-10 is involved in intestinal damage and mortality, independent of adaptive immunity, we analysed C. rodentium- infected Rag −/− and Il10 −/− Rag −/− recipients that were treated with IL-23p19 blocking or control antibodies. Il10 −/− Rag −/− recipients treated with control antibodies died between 5 and 10 days after infection; however, a neutralizing IL-23p19 antibody treatment rescued the survival of the infected mice ( Fig. 4d ). Furthermore, IL-23p19 antibody treatment prevented tissue damage at day 6 after infection compared with control antibodies ( Fig. 4e ). These data show that in the absence of IL-10 the innate immune response is unchecked, and excessive IL-23 contributes to early morbidity and death. To verify that blocking IL-23 also can reduce mortality in fully immune competent mice lacking only macrophage-derived IL-10, we analysed C. rodentium- infected Il10 flox/flox LysM-Cre mice, and as a control, Il10 flox/flox Cd4-Cre mice. Il10 flox/flox LysM-Cre mice treated with the isotype control antibody began to die at day 3 after infection, and none survived beyond day 11. However IL-23p19 antibody treatment had a significant effect on promoting the survival and preventing the epithelial cell damage of the infected Il10 flox/flox LysM-Cre mice ( Fig. 4f,g ). Altogether, these data indicate that macrophage-derived IL-10 plays a dominant role in controlling the amount of IL-23 production by macrophages in the large intestine during the early phases of C. rodentium infection, and IL-23 is responsible, at least in part, for morbidity and mortality and is a marker for the excessive response by innate immune cells. Gene signature of IL-10 competent large intestine macrophages Macrophages are heterogeneous, and therefore we determined which subset was responsible for preventing the excessive intestinal damage after C. rodentium infection. We reported previously that IL-10 competent GFP + cells in the large intestine from Il10 gfp reporter mice were mainly CD11b + , CD11c int and F4/80 + (ref. 11 ). Therefore we first gated GFP + or GFP − cells, then sorted IL-10 competent, GFP + CD11b + CD11c int F4/80 + macrophages (IL-10 + ) or their GFP − counterparts (IL-10 − ) from the large intestine of Il10 gfp reporter mice, and performed microarray analyses to obtain insight into their degree of relatedness ( Fig. 5a ). F4/80, CD11b and MHC class II expression levels in post sorted GFP + (IL-10 + ) and GFP − (IL-10 − ) populations were similar. While CD11c expression in the GFP − population had a broad distribution, we sorted those cells that had an amount of CD11c comparable to the GFP + population. Heatmap and MA plots showed that these two populations were closely related, with 242 mRNA transcripts that were differentially expressed ( Fig. 5b,c ). Two hundred and eleven genes were upregulated in the GFP + cells, including the cell surface markers, Vcam1, Cd209f and Cd163 . In addition, 31 genes, including Il12b , were downregulated ( Fig. 5c ). 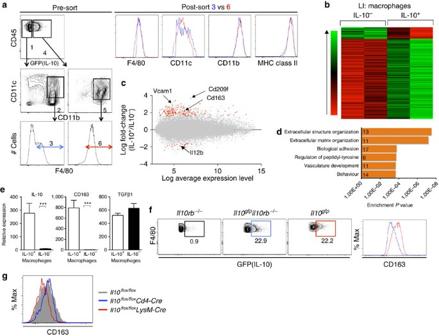Figure 5: Comparison of IL-10-producing and non-producing large intestinal macrophages. (a) Gating strategy for the microarray analysis of GFP+(IL10+) and GFP−(IL-10−) colonic lamina propria macrophages. Cells that were CD45+, MHC class II+, CD11b+, CD11cintand F4/80+were analysed. As depicted, the GFP−cells (gate #1) used to provide mRNA were the subset falling in gates #2 and #3, CD11b+, CD11cintand which were F4/80+(gate #3). The corresponding GFP+cells (gate #4) were less heterogeneous as they were almost entirely, CD11b+CD11cint(gate #5) and F4/80+(gate #6). After the sort, F4/80, CD11c, CD11b and MHC class II expressions of cells in gate 3 (blue) and gate 6 (red) were examined by flow cytometry. (b) Heatmap of differentially expressed probe sets (n=242) between IL-10+and IL-10−macrophages from the large intestine lamina propria (LI: macrophages) inIl10gfpreporter mice, ordered by average difference in intensity. LI, Large Intestine. (c) MA plot of all probe sets on the array. Red points significantly above zero represent higher expression in IL-10+macrophages compared to IL-10−macrophages (n=211), while points significantly below zero represent the inverse relationship (n=31). Grey points indicate probe sets that did not exhibit a significant difference in expression levels, according to criteria described in Methods. (d) Enriched Gene Ontology biological processes among upregulated genes, as determined by DAVID (e) IL-10+and IL-10−macrophages (CD11b+CD11cintF4/80+) were sorted from large intestine lamina propria ofIl10gfpreporter mice and analysed for expression ofIl10,Cd163andTgfβ1by real-time PCR. Data are presented relative to L32 expression and are presented as average and s.d. of two independent experiments. (f) (Left) GFP (IL-10) expression by colonic macrophages inIl10rb−/−,Il10gfpil10rb−/−andIl10gfpmice. Gated on CD45+MHC class II+CD11b+CD11cintF4/80+cells. (Right) CD163 expression by IL-10 positive macrophages inIl10gfpmice (red) and inIl10gfpil10rb−/−mice (blue). (g) CD163 expression in large intestinal macrophages (CD11b+CD11cintF4/80+cells) fromIl10flox/floxLysM-Cre(red),Il10flox/floxCd4-Cre(blue) andIl10flox/flox(grey) mice. Data are representative of one of the two independent experiments. Figure 5: Comparison of IL-10-producing and non-producing large intestinal macrophages. ( a ) Gating strategy for the microarray analysis of GFP + (IL10 + ) and GFP − (IL-10 − ) colonic lamina propria macrophages. Cells that were CD45 + , MHC class II + , CD11b + , CD11c int and F4/80 + were analysed. As depicted, the GFP − cells (gate #1) used to provide mRNA were the subset falling in gates #2 and #3, CD11b + , CD11c int and which were F4/80 + (gate #3). The corresponding GFP + cells (gate #4) were less heterogeneous as they were almost entirely, CD11b + CD11c int (gate #5) and F4/80 + (gate #6). After the sort, F4/80, CD11c, CD11b and MHC class II expressions of cells in gate 3 (blue) and gate 6 (red) were examined by flow cytometry. ( b ) Heatmap of differentially expressed probe sets ( n =242) between IL-10 + and IL-10 − macrophages from the large intestine lamina propria (LI: macrophages) in Il10 gfp reporter mice, ordered by average difference in intensity. LI, Large Intestine. ( c ) MA plot of all probe sets on the array. Red points significantly above zero represent higher expression in IL-10 + macrophages compared to IL-10 − macrophages ( n =211), while points significantly below zero represent the inverse relationship ( n =31). Grey points indicate probe sets that did not exhibit a significant difference in expression levels, according to criteria described in Methods. ( d ) Enriched Gene Ontology biological processes among upregulated genes, as determined by DAVID ( e ) IL-10 + and IL-10 − macrophages (CD11b + CD11c int F4/80 + ) were sorted from large intestine lamina propria of Il10 gfp reporter mice and analysed for expression of Il10 , Cd163 and Tgf β 1 by real-time PCR. Data are presented relative to L32 expression and are presented as average and s.d. of two independent experiments. ( f ) (Left) GFP (IL-10) expression by colonic macrophages in Il10rb −/− , Il10 gfp il10rb −/− and Il10 gfp mice. Gated on CD45 + MHC class II + CD11b + CD11c int F4/80 + cells. (Right) CD163 expression by IL-10 positive macrophages in Il10 gfp mice (red) and in Il10 gfp il10rb −/− mice (blue). ( g ) CD163 expression in large intestinal macrophages (CD11b + CD11c int F4/80 + cells) from Il10 flox/flox LysM-Cre (red), Il10 flox/flox Cd4-Cre (blue) and Il10 flox/flox (grey) mice. Data are representative of one of the two independent experiments. Full size image An annotation search in DAVID (database for Annotation, Visualization and Integrated Discovery functional classification tool) yielded unexpectedly enriched functional categories among upregulated genes in GFP + macrophages ( P <0.05), including: extracellular structure organization, extracellular matrix organization, biological adhesion, regulation of peptidyl-tyrosine, vasculature development and behaviour. However, no pathways were identified for the downregulated genes, likely reflecting the small number of genes with decreased expression ( Fig. 5d and Supplementary Fig. 6 ). We validated increased expression of Il10 and Cd163 in GFP + colonic macrophages by real-time reverse transcription PCR. In contrast, both the macrophage populations produced Tgfb1 mRNA ( Fig. 5e ). We also confirmed increased expression of CD163 in GFP + macrophages by flow cytometry ( Fig. 5f ). It has been reported CD163 is an IL-10 target gene in vitro [33] . Therefore we compared IL-10 receptor expression in IL-10 + and IL-10 − colonic macrophages. However there was no difference in receptor expression. To determine if IL-10 provides an autocrine signal in macrophages in vivo , we crossed Il10 gfp mice with Il10rb −/− mice. Interestingly, we found a similar frequency of GFP + colonic macrophages in mice that had not received any IL-10R signals in vivo ( Fig. 5f ). However, intestinal macrophages from Il10rb −/− mice showed reduced CD163 cell surface expression ( Fig. 5f ). To determine if an autocrine IL-10 signal could be responsible for the increased expression of CD163 by intestinal macrophages, we analysed cells from Il10 flox/flox LysM-Cre and control mice. Intestinal macrophages expressed increased CD163 in Il10 flox/flox Cd4-Cre and Il10 flox/flox mice compared with Il10 flox/flox LysM-Cre ( Fig. 5g ). These data suggest that autocrine IL-10 may play a role in the induction of the phenotype of the IL-10-producing colonic macrophage subset, but IL-10 signals, either autocrine or paracrine, are not required for the induction of IL-10 competence in these cells. IL-10 competent macrophages are protective To determine if the reporter positive subset of large intestinal macrophages is required for preventing the excessive inflammation after C. rodentium infection, we transferred sorted, reporter expressing GFP + (IL-10 + ) or GFP − (IL-10 − ) colonic macrophages from Il10 gfp mice into C. rodentium- infected Il10 −/− Rag −/− recipients ( Fig. 6a ). When GFP + (IL-10 + ) macrophages were transferred, we detected a marked increase in the survival and protection of tissue damage in the intestine compared with recipients of GFP − cells ( Fig. 6b ). Indeed we detected a significant reduction of inflammatory cell recruitment, including monocytes and granulocytes, in the large intestine of recipients of GFP + colonic macrophages after C. rodentium infection ( Fig. 6c ). Furthermore, chemokines potentially involved in the recruitment of monocytes and neutrophils to the large intestine, including CCL3, CCL4 and CCL5, were significantly decreased in the recipients of GFP + cells ( Fig. 6c ). These data show that IL-10 from macrophages in the large intestine is indispensable for limiting the excessive inflammation by regulating the inflammatory cell recruitment during the innate response. 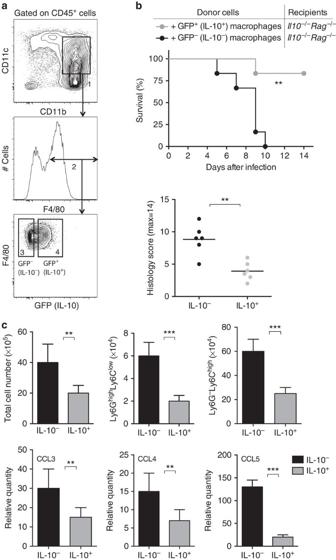Figure 6: IL-10 competent macrophages can rescue survival after infection. Il10−/−Rag−/−mice were infected withC. rodentium. On day 1 after infection, macrophages (CD11b+CD11cintF4/80+cells) were sorted from large intestine ofIl10gfpreporter mice and 5 × 105cells per mouse of GFP+(IL-10+) or GFP−(IL10−) populations were injected intravenously. (a) Gating strategy for obtaining GFP+(IL-10+) and GFP−(IL-10−) colonic macrophages for adoptive cell transfer. CD45+colonic lamina propria cells were selected on the basis of CD11b+, CD11cintexpression (gate #1) and F4/80 expression (gate #2) and further separated into GFP+(IL-10+) (gate #4) or GFP−(IL-10−; gate #3) populations. (b) Survival and histology score at day 6 after infection were monitored and is presented as a summary of two independent experiments with 3–5 mice per group. (c) (Top) total cell numbers were counted from large intestine at day 6 after infection. Frequencies of monocytes (Ly6G−Ly6Chigh) and granulocytes (Ly6GhighLy6Clow) were measured by flow cytometry and cell numbers were calculated according to the respective total cell number. Cell numbers are presented as averages and s.d. from three mice per group from two independent experiments. (Bottom) analysis ofCcl3, Ccl4andCcl5mRNA transcripts in the large intestine at day 6 after infection. Data are presented as averages with s.d. from three mice per group from two independent experiments. Student’st-test, **P<0.01, ***P<0.001. Figure 6: IL-10 competent macrophages can rescue survival after infection. Il10 −/− Rag −/− mice were infected with C. rodentium . On day 1 after infection, macrophages (CD11b + CD11c int F4/80 + cells) were sorted from large intestine of Il10 gfp reporter mice and 5 × 10 5 cells per mouse of GFP + (IL-10 + ) or GFP − (IL10 − ) populations were injected intravenously. ( a ) Gating strategy for obtaining GFP + (IL-10 + ) and GFP − (IL-10 − ) colonic macrophages for adoptive cell transfer. CD45 + colonic lamina propria cells were selected on the basis of CD11b + , CD11c int expression (gate #1) and F4/80 expression (gate #2) and further separated into GFP + (IL-10 + ) (gate #4) or GFP − (IL-10 − ; gate #3) populations. ( b ) Survival and histology score at day 6 after infection were monitored and is presented as a summary of two independent experiments with 3–5 mice per group. ( c ) (Top) total cell numbers were counted from large intestine at day 6 after infection. Frequencies of monocytes (Ly6G − Ly6C high ) and granulocytes (Ly6G high Ly6C low ) were measured by flow cytometry and cell numbers were calculated according to the respective total cell number. Cell numbers are presented as averages and s.d. from three mice per group from two independent experiments. (Bottom) analysis of Ccl3, Ccl4 and Ccl5 mRNA transcripts in the large intestine at day 6 after infection. Data are presented as averages with s.d. from three mice per group from two independent experiments. Student’s t -test, ** P <0.01, *** P <0.001. Full size image A balanced innate immune response is required for the protection from infection, and preventing excessive inflammation and tissue damage. Here we address what mediators control excessive inflammation and mortality during innate immune responses against mucosal bacteria, and the cell type and the mechanism responsible for the resolution of inflammatory response early during infection. IL-10 is a potent inhibitor of the production of TNF, IL-1, IL-6 and IL-12 in vitro [34] , [35] , and is therefore a good candidate for limiting the excessive inflammation in the intestinal mucosae. In the context of mucosal infectious disease, studies using Salmonella choleraesuis [15] , Klebsiella pneumoniae [16] , Listeria monocytogenes [18] and Candida albicans [19] have reported an increase in pathogen clearance, because the lack of IL-10 enhanced pro-inflammatory cytokines. In these situations the lack of IL-10 was beneficial to the host. In contrast, during infection with Toxoplasma gondii [17] , [21] , [22] and Trypanosoma cruzi [23] , infection in the absence of IL-10 caused excessive and often lethal inflammatory responses. These data highlight the importance of IL-10 in influencing the proper balance of innate immunity following infection with a variety of pathogens. We observed that C. rodentium was cleared slightly faster in mice deficient for IL-10, but these animals suffered from high morbidity and mortality, indicative of increased inflammation. A recent study, however, reported only a beneficial effect of the lack of IL-10 following C. rodentium infection [20] . The discordant findings could reflect the fourfold increased dose of bacteria we used, but more likely reflect aspects of the endogenous microbiota in different mouse colonies, as the virulence of C. rodentium is dependent on other components of the microbial flora [36] . By analysing mouse strains with T cell- or myeloid cell-specific deletion of IL-10, we could implicate macrophage IL-10 in limiting the destructive immune response. Consistent with this, intestinal tissue from Il10 flox/flox Cd4-Cre mice produced more IL-10 protein than tissue from Il10 flox/flox LysM-Cre mice, both at steady state and at early time points after infection, suggesting that macrophages are major IL-10-producing cells in the colon, both before and after bacterial infection. Indeed, colonic macrophages were GFP + before and after infection in Il10 gfp reporter mice. Macrophage IL-10 is indispensable for maintaining a balance in adaptive immune responses in the mucosae [11] , [37] , [38] , [39] , [40] , and here we demonstrate its importance during the innate immune response. It is possible, however, that IL-10-producing intestinal macrophages acquire inflammatory features during bacterial infection, or alternatively, that many intestinal macrophages can rapidly acquire the ability to produce IL-10. We showed that adoptive transfer of IL-10-producing intestinal macrophages from reporter mice, but not macrophage populations that did not express IL-10, rescued the survival of infected, IL-10-deficient mice. Therefore the GFP − colonic macrophages could not induce sufficient IL-10 production to attain a protective function during this acute infection. Although we have shown that IL-10 from colonic macrophages is protective, we cannot formally exclude the possibility that the GFP − cells were not protective because they could not home to the intestine or survive well after transfer. We consider this unlikely, because we did not see an increase in GFP + cells after infection. Therefore, while we suggest that the IL-10-producing intestinal macrophages could be a relatively stable subset; further experiments will be required to prove that this is the case. Interestingly, while the transcriptomes of the two colonic macrophage subsets are similar, the GFP + cells have increased expression of genes involved in extracellular matrix organization, vascular development, and others involved in tissue regeneration, such as the epidermal growth factor receptor and the platelet derived growth factor receptor. These data suggest that the GFP + macrophages may have a more prominent role in tissue homeostasis and repair. Here we have demonstrated that after a bacterial challenge the absence of IL-10 production by macrophages led to increased IL-23 synthesis, predominantly by macrophages, an enhanced innate immune response and fatal colitis. It is curious that IL-12 synthesis was not greatly affected, but indeed, it has been reported that IL-23 is associated with innate immune pathology in the intestine [41] , [42] . Consistent with this, IL-23 transgenic mice developed systemic inflammation that included the terminal ileum and colon, with infiltration of neutrophils and macrophages [43] . A few other studies have demonstrated that IL-10 negatively regulates IL-23 production, and therefore the absence of IL-10 caused an increase in IL-17-producing T cells and spontaneous intestinal inflammation [5] , [44] . We note, however, that the Il10 flox/flox LysM-Cre did not have increased IL-23 in the intestine at steady state nor did they spontaneously develop colitis. Our data demonstrate that exogenous IL-10 reduced in vitro IL-23 production by intestinal macrophages from C. rodentium- infected mice. In vivo , there is evidence that IL-10 acts directly on the IL-10-producing macrophage subset, although IL-10 competence did not depend on any IL-10 signals. IL-10-producing macrophages expressed increased CD163, however, which was dependent on IL-10R expression by these cells. Furthermore, GFP − macrophages from infected mice produced more IL-23p19 mRNA more than GFP + macrophages. However, in our analyses <40% of colonic macrophages were GFP + , and therefore the reduced inflammation and improved survival in wt mice suggests a paracrine role for IL-10 is also possible. Recent studies showed that IL-10 signals drive macrophages to express tolerogenic functions that prevent colitis [14] , [45] . However, those investigations focused on either steady-state or adaptive mucosal immune responses, not on innate mucosal immune responses, and they did not provide a mechanism or tie the protective role of IL-10 to macrophage IL-23 production. In humans, there is a study showing myeloid DCs from Crohn’s disease patients produced a higher amount of IL-23 and a lower amount of IL-10 after a bacterial stimulation when compared with ulcerative colitis patients [46] , leading us to propose that intestinal IL-10-producing myeloid cells might regulate IL-23 production not only in Crohn’s disease, but also in bacterial infection in humans. In summary, our data show that IL-10 synthesis by intestinal macrophages has a marked effect on regulating the innate immune response in mice through regulating macrophage IL-23 production after mucosal bacterial infection. Furthermore, intestinal macrophages are heterogenous, and although IL-10 competent and IL-10 − macrophages are similar, we suggest that they may not rapidly interconvert in vivo . Animals Mice were bred and housed under specific pathogen free conditions in the vivarium of the La Jolla Institute for Allergy & Immunology (LJI, La Jolla, CA). Eight weeks old female Il10 −/− , Il10rb −/− and Rag −/− mice were purchased from Jackson laboratory. Eight weeks old female Il10 gfp ( VertX ) mice were obtained from Christopher Karp (Cincinnati Children’s Hospital, OH) and also purchased from Jackson Laboratory. Il10 −/− Rag −/− mice were described previously [47] . Il10 flox/flox mice were obtained from Alexander Rudensky (Memorial Sloan-Kettering Cancer Center, NY) with the permission of Axel Roers (Dresden University of Technology, Germany). Il10 flox/flox mice were bred to Cd4-Cre , LysM-Cre and Cd11c-Cre mice, which were all purchased from Jackson laboratory. All mouse strains were generated on the C57BL6/J background or backcrossed at least 10 generations. All procedures were approved by the LJI Animal Care and Use Committee. C. rodentium infection A chloramphenicol-resistant variant of the wt C. rodentium strain DBS100 was cultured as previously described [30] . In brief, bacteria were cultured for 15–16 h in Luria-Bertani broth at 37 °C. Mice were infected with 2–3 × 10 9 CFU C. rodentium by oral gavage. In some experiments functional grade IL23p19 (G23-8) antibody or control rat IgG were injected intravenously at 100 μg per mouse at the time of infection. Antibodies were purchased from eBiosciences (San Diego, CA). GFP + (IL-10 + ) and GFP − (IL-10 − ) macrophages were sorted from colon tissue of uninfected Il10 gfp (VertX) mice as CD45 + , MHC class II + , CD11b + , F4/80 + , CD11c int cells. One day after infection, 5 × 10 5 macrophages were injected intravenously per mouse. For CFU determination, the faecal pellets and the spleen were weighed, homogenized and plated on chloramphenicol-containing MacConkey agar plates in serial dilutions. FITC-dextran permeability assay In vivo permeability assays to assess intestinal barrier function were performed using fluorescein isothiocyanate (FITC)-labelled dextran (Sigma) as described previously [30] . In brief, mice were infected with C. rodentium . At day 0 or 6 after infection, mice were gavaged with FITC-dextran (60 mg per 100 g body weight) and serum was collected retro-orbitally 4 h later. Blood cells in serum samples were removed and the fluorescence intensity of FITC-dextran was measured. FITC-dextran concentrations were determined from the standard curves generated by serial dilution. Reagents and antibodies For flow cytometry and cell sorting the following antibodies were used: CD11b (M1/70), CD11c (N418), F4/80 (BM8), CD45 (30-F11), IA/IE (M5/114.15.2), Ly6C (HK1.4), Ly6G (1A8), CD4 (RM4–5), TCRβ (H57–597), CD163 (polyclonal). Antibodies were purchased from BD Biosciences (San Diego, CA), eBiosciences (San Diego, CA), BioLegend (San Diego, CA) or Antibodies-online.com. Cell sorting was performed on an Aria II instrument (BD Biosciences). Cytokines and chemokines were quantified using either the Bio-plex multicytokine assay (Bio-Rad, Hercules, CA), as described previously [48] , IL-23p19, IL-22 or IL-12p70 ELISA kits (eBiosciences, San Diego, CA) or a IL-6 ELISA kit (BD, San Diego, CA). Colon fragment cultures Large intestines were harvested and 3-mm colon fragments were cultured for 24 h in DMEM with 10% FBS and antibiotics. Supernatants were analysed for cytokines and chemokines in ratio to the weight of the corresponding tissue fragment. Isolation of lamina propria cells Large intestines were harvested, opened longitudinally and washed to remove faecal content. Intestines were cut into small pieces and incubated in a horizontal shaker at 37 °C in the presence of 2.5 mM EDTA three times for 20 min to remove epithelial cells. Colon pieces were minced and digested for 20 min with 1 mg ml −1 Collagenase type VIII (Sigma, St Louis, MO) at 37 °C. Lamina propria cells were filtered and stained for flow cytometric analysis or cell sorting. Histology Tissue sections were taken from the middle colon and fixed in 10% formalin. After embedding in paraffin, 5-μm sections were cut and stained with hematoxylin-eosin. Histological scores were assigned in a blinded manner according to the following criteria: (i) mucosal architecture (0, normal; 1, focally abnormal; 2, diffusely abnormal; 3, severely abnormal); (ii) inflammatory cell infiltration of mucosa (0, normal; 1, mild infiltration; 2, moderate infiltration; 3, severe infiltration), submucosa (0, normal; 1, mild infiltration; 2 moderate infiltration; 3, severe infiltration), muscle (0, normal; 1 moderate to severe) and serosa (0, absent; 1, present); (iii) epithelial erosions and ulcerations (0, absent; 1, present); (iv) crypt abscesses (0, absent; 1, present); and (v) goblet cell loss (0, absent; 1, present). The maximal total score for colitis severity is 14. Relative mRNA quantification Total RNA was extracted from sorted cells or 2–3-mm long colon tissue fragments using the RNeasy Mini kit (Qiagen, Hilden, Germany) according to the manufacturer's instructions. Genomic DNA was digested with DNase I (Qiagen), cDNA was synthesized using iScript (Bio-Rad, Hercules, CA) and real-time PCR was performed using SYBRgreen (Roche, Indianapolis, IN) on a LightCycler instrument (Roche). The primers were as follows: L32, 5′-GAA ACT GGC GGA AAC CCA-3′ (sense), 5′-GGA TCT GGC CCT TGA ACC TT-3′ (antisense), CD163, 5′-GGT GGA CAC AGA ATG GTT CTT C-3′ (sense), 5′-CCA GGA GCG TTA GTG ACA GC-3′ (antisense), TGFβ1, 5′-ACC ATG CCA ACT TCT GTC-3′ (sense), 5′-CGG GTT GTG TTG GTT GTA GA-3′ (antisense), Il10 , 5′-GCC ACA TGC TCC TAG AGC TG-3′ (sense), 5′-CAG CTG GTC CTT TGT TTG AAA-3′ (antisense), Il23p19 , 5′-AAT AAT GTG CCC CGT ATC CA-3′ (sense), 5′-GGA TCC TTT GCA AGC AGA AC-3′ (antisense), Il12p35 , 5′-GTG AAG ACG GCC AGA GAA A-3′ (sense), 5′-GGT CCC GTG TGA TGT CTT C-3′ (antisense), Il12p40 , 5′-AGC AGT AGC AGT TCC CCT GA-3′ (sense), 5′-AGT CCC TTT GGT CCA GTG TG-3′ (antisense). Microarray data processing and analysis All microarray data sets were processed in R, using customized scripts and Bioconductor modules [49] . Raw intensity data were normalized with the ‘rma’ function, with default parameters. Differential expression analysis was performed using the ‘limma’ package. Probe sets were deemed significantly differentially expressed only if their corrected P values were <0.05 and the difference was at least threefold. Heatmaps containing the differentially expressed genes in each set were built using the ‘regHeatmap’ function of the ‘Heatplus’ module and sorted by average fold change. The 242 probe sets that were significantly differentially expressed were mined for enriched Gene Ontology biological process terms using DAVID ( http://david.abcc.ncifcrf.gov ). Immunofluorescence Colons and ilea were harvested, flushed with PBS(Life Technologies, Carlsbad, CA) and fixed with 4% paraformaldehyde (Electron Microscopy Sciences, Hatfield, PA) in PBS overnight at 4 °C and then equilibrated in 30% w/v sucrose solution in PBS for another 24 h. Tissues were briefly washed in PBS, frozen in OCT and stored at −80 °C. Cryostat sections were cut at 16-μm thickness and air-dried for 30 min. Sections were rehydrated for 10 min in PBS and nonspecific binding sites were saturated with 10% normal goat serum, 0.5% bovine serum albumin (both from Gemini Bio-Products, West Sacramento, CA) in the presence of 0.1% Triton X-100 in PBS for 1 h. Tissues were incubated with anti-F4/80 rat monoclonal antibodies (50 μg ml −1 , BM8, eBiosciences) and anti-GFP rabbit antiserum (5 μg ml −1 , ab290, Abcam, Boston, MA) overnight at 4 °C. Following washing, sections were reacted with donkey anti-rat DyLight 549-labelled (1.4 μg ml −1 , Jackson Immunoresearch) and goat anti-rabbit F(ab')2 fragment Alexa Fluor 647-labelled secondary antibodies (4 μg ml −1 , Invitrogen) for 1 h at room temperature. Slides were washed, mounted in Prolong Gold antifade reagent (Invitrogen) with a cover slip and examined with FluoView FV10i confocal microscope (Olympus). Imaging was performed at room temperature, using 60 × /1.35 NA oil objective. To improve feature visibility images were processed by contrast stretching using identical procedures. Statistical analysis The Student’s t -test was used for statistical analysis except for the survival and histological scores, for which the log-rank test and the Mann–Whitney test were used, respectively. Differences were considered significant at P <0.05. Accession codes. Microarray data has been deposited in the Gene Expression Omnibus (GEO) database under accession code GSE58677 . How to cite this article: Krause, P. et al . IL-10-producing intestinal macrophages prevent excessive antibacterial innate immunity by limiting IL-23 synthesis. Nat. Commun . 6:7055 doi: 10.1038/ncomms8055 (2015).